Topologically protected quantum state transfer in a chiral spin liquid Topology plays a central role in ensuring the robustness of a wide variety of physical phenomena. Notable examples range from the current-carrying edge states associated with the quantum Hall and the quantum spin Hall effects to topologically protected quantum memory and quantum logic operations. Here we propose and analyse a topologically protected channel for the transfer of quantum states between remote quantum nodes. In our approach, state transfer is mediated by the edge mode of a chiral spin liquid. We demonstrate that the proposed method is intrinsically robust to realistic imperfections associated with disorder and decoherence. Possible experimental implementations and applications to the detection and characterization of spin liquid phases are discussed. The decoherence of both quantum states and quantum channels represents a major hurdle in the quest for the realization of scalable quantum devices [1] , [2] . Several avenues are currently being explored to address these important challenges. For example, quantum error correction can significantly extend the lifetime of quantum memories and suppress the errors associated with quantum logic operations [3] , [4] ; its practical realization, however, requires a high level of quantum control that is as yet, not experimentally accessible. Topology also provides a paradigm for achieving protected quantum states; indeed, if such states can be stored in the topological degrees of freedom of certain exotic states of matter, they become intrinsically robust against local noise [5] , [6] . Alternatively, the implementation of long-lived quantum memories can be achieved by encoding quantum bits in carefully chosen physical degrees of freedom. In particular, the natural isolation of nuclear spins immunizes them from the environment and makes them an exceptional candidate for the storage of quantum information [7] , [8] , [9] , [10] , [11] . This isolation implies, however, that spatially remote memories interact extremely weakly; this shifts, the challenge of scalability to the development of quantum channels capable of connecting remote registers in a robust and noise-free manner. Here we describe a novel approach to the realization of intrinsically robust quantum channels, which enable state transfer between remote qubit registers. We envision state transfer to be mediated by a two-dimensional (2D) system composed of interacting qubits (for example, spins or pseudo-spins); specifically, the system is tuned into a gapped chiral spin liquid phase that harbours a fermionic edge mode. The prototype of such a spin liquid is the gapped B phase (CSLB) of the Kitaev honeycomb model [12] . Although such a phase is best known for its non-Abelian vortex excitations, here, by operating at finite temperatures below the gap, we make use of its Majorana fermionic edge mode as a topologically protected quantum channel. By contrast to previous spin-chain-based approaches, which are critically sensitive to disorder [13] , [14] , our method exploits topological protection to enable high-fidelity quantum information transport. We will discuss possible applications of our protocol for the spectroscopic characterization of spin liquid states [15] . Finally, we describe an example implementation based upon an engineered superconducting qubit lattice. Approach to topologically protected state transfer Our approach to quantum state transfer is schematically illustrated in Fig. 1 . Quantum information is encoded in a two-qubit register, with each qubit capable of being individually manipulated. The register is coupled to the edge of a 2D droplet, whose elements we assume cannot be individually addressed but can be globally ‘engineered’ to create a spin liquid state in the CSLB phase. The transfer protocol proceeds by mapping the quantum information stored in the left-hand spin-register onto the chiral edge mode of the droplet. The resulting wavepacket traverses the edge before retrieval at the remote register. 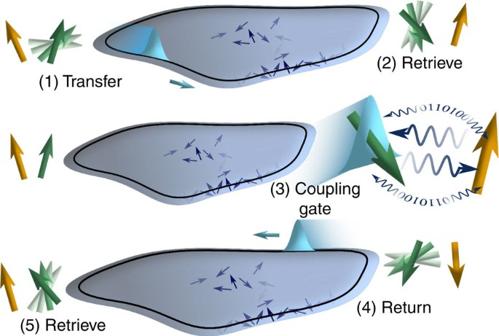Figure 1: Schematic representation of topologically protected state transfer. The grey droplet represents a 2D array of interacting qubits (spins or pseudo-spins) tuned into the CSLB phase. Quantum registers composed of a transfer qubit (green) and a memory qubit (gold) are arranged around the edge of the 2D droplet and coupling between them occurs through the chiral edge mode. (1) By mapping the quantum information onto a fermionic wavepacket (blue) travelling along the edge, the quantum state can be transferred to a remote register. The wavepacket travels only in the direction of the blue arrow; this chirality prevents mode localization and destructive backscattering. At a specified time at the remote register location, the coupling is turned on and the wavepacket is captured (2). Given an ancillary memory qubit and local register manipulations, a two-qubit gate (3) can be performed before the quantum state is transferred back to the original register and stored (4–5). This allows for universal computation between the memory qubits of spatially separated registers. Figure 1: Schematic representation of topologically protected state transfer. The grey droplet represents a 2D array of interacting qubits (spins or pseudo-spins) tuned into the CSLB phase. Quantum registers composed of a transfer qubit (green) and a memory qubit (gold) are arranged around the edge of the 2D droplet and coupling between them occurs through the chiral edge mode. (1) By mapping the quantum information onto a fermionic wavepacket (blue) travelling along the edge, the quantum state can be transferred to a remote register. The wavepacket travels only in the direction of the blue arrow; this chirality prevents mode localization and destructive backscattering. At a specified time at the remote register location, the coupling is turned on and the wavepacket is captured (2). Given an ancillary memory qubit and local register manipulations, a two-qubit gate (3) can be performed before the quantum state is transferred back to the original register and stored (4–5). This allows for universal computation between the memory qubits of spatially separated registers. Full size image A distinct feature of our protocol, as compared with previous approaches [13] , [14] , [16] , is the fundamental robustness of the quantum channel. The chiral nature of the Majorana fermionic edge mode ensures that destructive backscattering during state transfer is highly suppressed. The characteristic (linear) dispersion of the edge-mode also ensures that wave packet distortion is minimized. Moreover, we demonstrate that our approach is remarkably insensitive to disorder and decoherence affecting both the bulk and edge of the droplet. Although any spin system with a stable CSLB-like phase can potentially mediate topologically protected state transfer (TPST), to illustrate the microscopic mechanism responsible for such state transfer, we turn initially to a particular model and will later generalize our analysis to include the effects of disorder, additional interactions and decoherence. TPST on the decorated honeycomb We now consider a specific exactly solvable model, which supports robust TPST [17] . Within the so-called Yao-Kivelson model, the spin (or pseudo-spin) 1/2 particles are situated on a triangular-decorated honeycomb lattice as depicted in Fig. 2 (ref. 17 ). 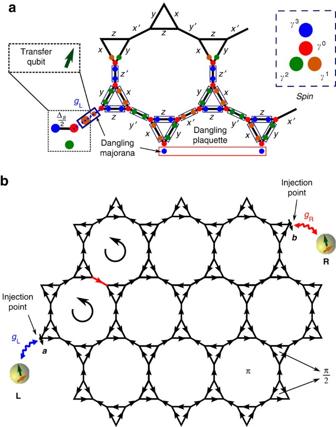Figure 2: Coupling between qubit register and the droplet edge. (a) Schematic representation of the generalized Kitaev Hamiltonian on the decorated honeycomb lattice. Spins are represented by four Majorana operators; spin–spin interactions become products of the four Majoranas living on each link. Boxed spins correspond to theoperators, which determine the effective hopping associated with theγ0Majoranas. Coupling (dashed line) between the quantum register and the 2D droplet can occur at any edge vortex with an unpaired Majorana; the Majorana flavour determines the form of the spin–spin interaction that introduces the desired additional hopping. (b) Schematic representation of the ground state flux configuration. Each arrow represents a Majorana hopping ofi, yieldingπphase (oriented counterclockwise) around the dodecagonal plaquettes andπ/2 phase around the triangular plaquettes. Vortex excitations (circular arrows) correspond to the flipping of aUijlink (red arrow and link), which yieldsw(p)=−1 in the two adjacent plaquettes. Quantum registers corresponding to a transfer qubit (green) and a memory qubit (gold) are shown coupled into the droplet (injection points) at two different dangling edge spins. The associated Hamiltonian naturally generalizes the Kitaev model [12] and features a chiral spin liquid ground state (CSLB phase), Figure 2: Coupling between qubit register and the droplet edge. ( a ) Schematic representation of the generalized Kitaev Hamiltonian on the decorated honeycomb lattice. Spins are represented by four Majorana operators; spin–spin interactions become products of the four Majoranas living on each link. Boxed spins correspond to the operators, which determine the effective hopping associated with the γ 0 Majoranas. Coupling (dashed line) between the quantum register and the 2D droplet can occur at any edge vortex with an unpaired Majorana; the Majorana flavour determines the form of the spin–spin interaction that introduces the desired additional hopping. ( b ) Schematic representation of the ground state flux configuration. Each arrow represents a Majorana hopping of i , yielding π phase (oriented counterclockwise) around the dodecagonal plaquettes and π /2 phase around the triangular plaquettes. Vortex excitations (circular arrows) correspond to the flipping of a U ij link (red arrow and link), which yields w ( p )=−1 in the two adjacent plaquettes. Quantum registers corresponding to a transfer qubit (green) and a memory qubit (gold) are shown coupled into the droplet (injection points) at two different dangling edge spins. Full size image where are Pauli spin operators ( ). The model may be solved by introducing four Majorana operators, { γ 0 , γ 1 , γ 2 , γ 3 } for each spin, as shown schematically in Fig. 2a and by representing the spin algebra as: σ x = iγ 1 γ 0 , σ y = iγ 2 γ 0 , σ z = iγ 3 γ 0 (refs 12 , 17 ). The Majorana operators are Hermitian and satisfy the standard anticommutation relation { γ l , γ m }=2 δ lm . The Hilbert space associated with the physical spin is a 2D subspace of the extended 4D Majorana Hilbert space; thus, we must impose the gauge projection, P =(1+ D )/2, where D = γ 1 γ 2 γ 3 γ 0 (ref. 12 ). Transforming to Majorana operators results in the extended Hamiltonian where ( α depends on the type of ij -link) for ij connected and zero otherwise; these correspond to the boxed Majorana pairs illustrated in Fig. 2a . Remarkably each commutes with the Hamiltonian and with all other , implying that the extended Hilbert space can be divided into sectors corresponding to static choices of { U i , j =±1} (refs 12 , 17 ). The choice of { U i , j } yields a Hamiltonian, which is quadratic in the γ 0 Majorana operators; from the perspective of these Majoranas, U i , j is a static background gauge field. The physical states are sensitive only to the flux of the gauge field, , where p represents a plaquette, ∂ p is its boundary and ij is oriented according to the arrows in Fig. 2b (ref. 17 ). For any link with U i , j =+1, this orientation can also be interpreted as the direction in which a γ 0 Majorana hops in order to accumulate a π /2 phase. The ground state flux sector of the model has w ( p )=+1 for all plaquettes, corresponding to π phase around the dodecagonal plaquettes and π /2 phase around the triangular plaquettes, as shown in Fig. 2b . The π /2 phase around the triangular plaquettes indicates the breaking of time-reversal symmetry necessary for a chiral ground state. Alternate flux sectors contain plaquettes with vortex excitations defined by w ( p )=−1. In general, such vortices are energetically gapped by Δ v , but the energy and dynamics of vortices near the edge are controlled by the details of the boundary. In each flux sector, the associated Majorana Hamiltonian can be diagonalized through a unitary transformation Q, such that , yielding , where , N is the number of spins on the lattice and the index k is ordered according to energy. Owing to particle-hole symmetry, ɛ k =− ɛ − k and ; thus, by restricting to k >0, where c k and satisfy Dirac anticommutation relations. Diagonalization of the ground state flux sector on a cylinder yields three bulk fermion bands, energetically gapped by Δ b , as shown in Fig. 3 (ref. 17 ). At the edge, the fermionic quasiparticles form gapless chiral modes, which are guaranteed by the nontrivial Chern number of the bulk fermion bands. 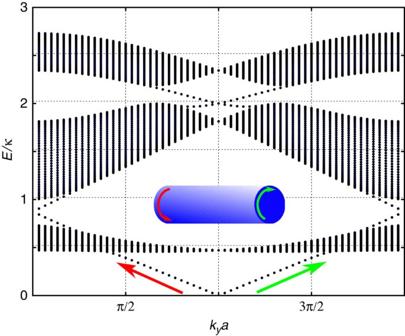Figure 3: Fermionic spectrum of the ground state flux sector. The model is placed on a cylinder of circumference 61 and width 40 unit cells, with a zigzag edge oriented such that theydirection is periodic55. The chiral edge modes are clearly visible nearkya=πat energies below the bulk fermion gap Δb=0.46κ. Numerical simulations also indicate the following values of the two vortex gaps: 0.14κ (dodecagonal vortex) and 0.17κ (triangular vortex). The inset illustrates the oppositely propagating chiral edge mode (red and green) at each end of the cylinder. In a droplet, the flux sector with completely opposite flux in each plaquette would support edge modes travelling in a reversed orientation. Figure 3: Fermionic spectrum of the ground state flux sector. The model is placed on a cylinder of circumference 61 and width 40 unit cells, with a zigzag edge oriented such that the y direction is periodic [55] . The chiral edge modes are clearly visible near k y a = π at energies below the bulk fermion gap Δ b =0.46κ. Numerical simulations also indicate the following values of the two vortex gaps: 0.14κ (dodecagonal vortex) and 0.17κ (triangular vortex). The inset illustrates the oppositely propagating chiral edge mode (red and green) at each end of the cylinder. In a droplet, the flux sector with completely opposite flux in each plaquette would support edge modes travelling in a reversed orientation. Full size image Qubit coupling to a chiral edge We now consider the addition of qubit registers, which can be individually manipulated and read out, to the edge of the exactly solved model with open boundary conditions [18] . Each edge spin with coordination two has an uncoupled Majorana operator, which we term dangling as depicted in Fig. 2a . We can extend the definition of vortices to include the dangling plaquettes defined by the U i , j links between dangling Majoranas, as shown by the red rectangle in Fig. 2a . These dangling vortices are completely decoupled from the fermions and lead to a large degeneracy of the model. However, generic perturbations will lift this degeneracy by gapping out these dangling vortex states; in this situation, as we later describe, the control of dangling vortices at the injection point will become important. To illustrate TPST, we consider the full Hamiltonian H T = H 0 + H int , where H int characterizes the coupling between the two spin registers (termed L and R ) and dangling spins at the edge of the droplet ( Fig. 2b ), Here, Δ S is the splitting of the register states (for example, by an applied field), β , η are chosen to respect the interaction symmetry at the injection points, and g L , g R represent the interaction strength between the registers and the injection spins ( a and b ) as shown in Fig. 2 . Transforming to Majorana operators yields , where, without loss of generality, we have chosen a σ x σ x register-edge interaction. The existence of a dangling Majorana at the droplet edge is critical to enable coupling to the edge mode. At the injection points ( Fig. 2b ), the register-edge coupling of equation (4) not only creates a fermionic excitation, but also introduces a dangling vortex (by flipping the U i , j corresponding to the adjacent dangling plaquette). Thus, in order to exploit the chiral fermion mode to transport quantum information, we will need to control the injection point ( Supplementary Fig. S1 ). Imperfections in such control will result in the spin-register coupling to additional nearby spins. However, as the nearest spins surrounding the injection point will not contain dangling Majoranas, these additional interactions will naturally gap out. Even in the presence of the additional interactions prescribed in equation (4), as U L,a and U R,b are conserved, the model remains exactly solvable. Expressed in terms of the eigenmodes of the unperturbed Hamiltonian in the ground state flux sector, where we have defined and ; in this language, the σ z spin state of the L(R) qubit is encoded in the occupation of the L(R) fermion mode. The first term of the Hamiltonian characterizes the modes of the 2D droplet, the second and third terms characterize the splitting associated with the spin registers, whereas the final two terms capture the coupling between the registers and the dangling edge spins. This Hamiltonian acts in the extended fermionic Hilbert space and returning to physical spin states requires gauge projection ( Supplementary Discussion ). TPST in the dot and droplet regime The coupling between the register and the chiral edge mode can be analysed in two distinct regimes: (1) the mesoscopic dot regime and (2) the macroscopic droplet regime. The distinction between these two regimes is best understood from a perspective of resolvability; in the dot regime, we consider the coupling to a small finite-size system, enabling energy resolution of the individual chiral edge modes. Thus, TPST is mediated by a single fermionic eigenmode of the system [14] . Meanwhile, in the droplet regime, we consider the coupling to a larger system, in which energy resolution at the single mode level would be extremely difficult. In this regime, we encode the spin register’s quantum information in a travelling fermionic wavepacket. In both the dot and droplet regimes, TPST relies on the coherent transfer of fermionic occupation from register L to R. In order for this to be well defined, we choose Δ S >0 and g L , g R <Δ S so that the effective Dirac fermions, , are conserved. In the dot regime, TPST can be understood by tuning Δ S to be resonant with a single-edge mode, , with energy ; so long as the coupling strength is weak enough to energetically resolve this mode, evolution is governed by the effective Hamiltonian, and hence, state transfer proceeds via resonant fermion tunnelling, as depicted in Fig. 4a (ref. 14 ). The timescale, τ , required to achieve high-fidelity state transfer depends only on the energy spacing between adjacent modes, , where is the system’s linear dimension; to prevent the leakage of quantum information into off-resonant fermionic modes, (ref. 14 ). 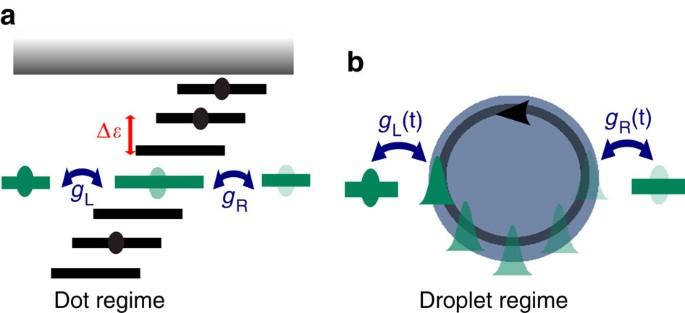Figure 4: Regimes of TPST. (a) Schematic representation of the dot regime, wherein TPST becomes analogous to tunnelling. In this mesoscopic dot regime, the coupling strength is kept weak enough to enable resolution of single-edge modes. (b) Schematic representation of the droplet regime, wherein TPST is achieved by mapping the quantum information from a spin register onto a travelling fermionic wavepacket. The wavepacket is caught at the remote register, after which a two-qubit gate (Supplementary Fig. S2) is performed before the information is returned (via a wavepacket) to the initial register. Figure 4: Regimes of TPST. ( a ) Schematic representation of the dot regime, wherein TPST becomes analogous to tunnelling. In this mesoscopic dot regime, the coupling strength is kept weak enough to enable resolution of single-edge modes. ( b ) Schematic representation of the droplet regime, wherein TPST is achieved by mapping the quantum information from a spin register onto a travelling fermionic wavepacket. The wavepacket is caught at the remote register, after which a two-qubit gate ( Supplementary Fig. S2 ) is performed before the information is returned (via a wavepacket) to the initial register. Full size image In the droplet regime, we encode the fermionic occupation into the presence/absence of a wavepacket travelling along the chiral edge, as illustrated in Fig. 4b (ref. 19 ). Upon tuning both spin registers to an energy Δ S , the encoding can be performed by choosing g L ( t ) with the following time dependence, where f ( t ) characterizes the shape of the desired wavepacket and v is the group velocity of the chiral mode. Subsequent retrieval can be similarly achieved by using time-reversal symmetry to appropriately choose the shaping of g R ( t ) ( Supplementary Methods ). We note that such wavepacket encoding is in direct analogy to the storage and retrieval of photonic wavepackets [20] , [21] , [22] . In contrast to the dot regime, the magnitude of the coupling strengths may be of order Δ S , which is independent of . However, the time scale of TPST includes the wavepacket’s propagation time, which depends on both the physical separation of the registers and the wavepacket group velocity. Effects of imperfections, disorder and decoherence Having explicitly demonstrated TPST in an exactly solvable model, we now consider additional imperfections, disorder, temperature and decoherence. As the CSLB phase has a bulk gap and a topological invariant protecting its chiral edge mode, we expect the effective low-energy fermion dynamics to be insensitive to small perturbations [12] . Furthermore, the chirality of the edge mode prevents localization and the Majorana nature of the edge fermions strongly suppresses the phase space for scattering, thereby limiting nonlinear corrections to the dispersion [13] , [14] , [16] . In the following, we consider various classes of imperfections arising from local spin perturbations and coupling to a finite temperature bath; these result in: (1) vortex excitations, (2) finite Majorana lifetime and (3) dynamical decoherence. At low temperatures T , there will be a dilute gas of bulk vortices, , where n p represents the total number of bulk plaquettes. As a vortex excitation corresponds to a π flux relative to the ground state, a circumambulating fermion acquires an additional phase of N v π . Thus, the presence of vortices can have two relevant effects: (1) vortices within a localization length, ξ ∼ a (where a is the lattice spacing), of the edge can scatter a travelling fermion and (2) an odd number of vortices induces a π -shift of the net phase [23] . Perturbations also generically lift the aforementioned degeneracy associated with dangling edge vortices. However, this will only affect the fidelity of TPST at the injection point, where one must ensure the existence of a single dangling edge Majorana. Away from the injection point, three possibilities arise: First, zero energy dangling vortices are completely decoupled from the fermions, and hence will be irrelevant for TPST. Second, low-energy dangling vortices will scatter only minimally, as the interaction strength between the dangling Majoranas, and hence the hopping strength across the dangling link, will be extremely weak (see Methods for details). Finally, much as in the bulk, the effect of high-energy dangling vortices will be suppressed by their gap. As static effects, all of the aforementioned error contributions can be abrogated by the use of tomography; hence, it is crucial to effectively freeze out vortex fluctuations on the time scale of TPST, and this is most easily accomplished at temperatures that are small compared with Δ v . Next, we consider the addition of generic perturbative local spin interactions, H p , to the full Hamiltonian, H T . Certain classes of perturbations leave the model exactly solvable; more generally, however, if H p is longer ranged or does not respect the model’s interaction symmetry, the gauge field acquires dynamics and the effective fermionic theory is no longer free. In order to understand these effects, we turn to a low-energy continuum theory of the Majorana edge (assuming that dangling vortex excitations are either decoupled or gapped out), where is the subset of in equation (3), which creates an edge excitation at momentum p and where we have switched to a continuum normalization of the Majorana field, { γ ( x ), γ ( y )}= δ ( x − y ) (ref. 23 ). The introduction of interactions induces decay of the quasiparticle excitations . This quasiparticle lifetime limits the size of the droplet around which coherent excitations may be sent. The leading order symmetry-allowed interaction is of the form [24] where λ characterizes the strength of the interaction. We estimate the decay rate of a single quasiparticle excitation using Fermi’s golden rule (see Methods for details). In the low-temperature limit ( ɛ p ≫ k B T ), To relate to the microscopic model parameters, we consider generic vortex-inducing local spin perturbations of strength κ ′, which yield in second-order perturbation theory. Substituting into equation (10) allows us to re-express the zero temperature decay rate as , where Δ S = vp is the energy of the injected TPST fermion. The surprisingly strong dependence on momenta suggests that quasiparticle decay can safely be neglected so long as p <1/ a . Finally, we consider dynamical decoherence due to weak coupling with a low-temperature phonon bath, which induces additional decay of the fermion involved in TPST. We assume that the bath couples to local spin operators and that its effect is characterized by its noise spectral density, (ref. 25 ). Multi-spin perturbations can be analysed in an analogous manner and do not change the qualitative results summarized below. In the bulk, each such operator creates a pair of vortices ( Fig. 2b ) in addition to creating or destroying a Majorana quasiparticle. As the fermionic edge modes are exponentially localized, the contribution of this process to the decay rate is suppressed by e − d /ξ , where d is the distance from site i to the edge. Moreover, there is an additional energy suppression from where ω 0 =2Δ v is the energy cost of creating a pair of vortices. This brings us to the primary decoherence effect: edge noise. There are two types of spin operators acting on the lattice edge: (1) those which only create or destroy an edge fermion (type I) and (2) those which also introduce vortices (type II–IV), as shown in Fig. 5 . Type I spin operators can only induce decay if they directly annihilate the injected TPST edge fermion, a process costing energy Δ S . By contrast, once a vortex is created at any edge plaquette it can scatter the travelling TPST fermion, implying that the associated decoherence is enhanced by a factor of , as depicted in Fig. 5 . 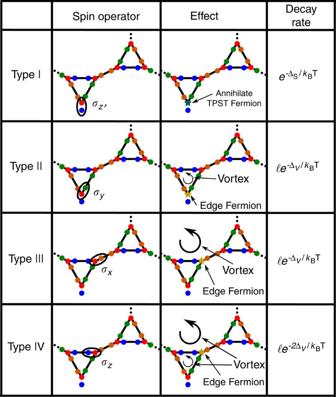Figure 5: Schematic representation of the various forms of edge decoherence. Type I spin operators correspond to non-vortex-inducing decoherence and can affect TPST only by annihilating the TPST fermion (teal star), a process suppressed by, where ΔSrepresents the detuning of the spin registers and hence, also the energy of the injected quasiparticle. Type II–IV spin operators create vortices (circular arrow) in edge plaquettes. Once a vortex is created at any edge site, it can scatter the travelling TPST fermion, leading to the decoherence being enhanced by(the droplet’s linear dimension). In addition to creating vortices, type II–IV spin operators also create un-gapped edge fermions (gold star), which we assume does not affect TPST, as quasiparticle interactions have been shown to be extremely weak. Thus, the total TPST decay rate induced by edge noise is, Figure 5: Schematic representation of the various forms of edge decoherence. Type I spin operators correspond to non-vortex-inducing decoherence and can affect TPST only by annihilating the TPST fermion (teal star), a process suppressed by , where Δ S represents the detuning of the spin registers and hence, also the energy of the injected quasiparticle. Type II–IV spin operators create vortices (circular arrow) in edge plaquettes. Once a vortex is created at any edge site, it can scatter the travelling TPST fermion, leading to the decoherence being enhanced by (the droplet’s linear dimension). In addition to creating vortices, type II–IV spin operators also create un-gapped edge fermions (gold star), which we assume does not affect TPST, as quasiparticle interactions have been shown to be extremely weak. Full size image Strikingly, the sources of decoherence in TPST are exponentially suppressed in temperature and thus can be controlled [14] . The above analysis generalizes to other types of noise sources. Of particular relevance in the context of solid-state spin systems are nuclear spin baths, in which , where t c is the bath’s correlation time. In this model, the Arrhenius-type energy suppressions of equation (11) becomes if (ref. 25 ). We now illustrate these considerations by discussing a specific implementation of our proposed technique. As a first example, let us consider an implementation of the robust quantum channel based upon the pseudo-spin degrees of freedom of superconducting qubits [26] , [27] , [28] . Specifically, we consider an engineered lattice of superconducting (SC) qubits tuned to the CSLB phase; the three distinct types of nearest neighbour interactions σ x σ x , σ y σ y , σ z σ z can be achieved, respectively, via a mutual inductance, an LC oscillator and a capacitance [28] , [29] . Such an approach could provide a superconducting pseudo-spin-edge quantum channel with remarkable properties. Specifically, the gapped nature of the CSLB phase strongly suppresses the effects of decoherence (Γ 0 ) typically associated with single SC-qubits. We will work with experimentally realistic parameters: temperature T ∼ 10 mK, a macroscopic length scale mm, κ ∼ 10 GHz, Δ S ∼ 0.8 GHz, Δ V ∼ 1.7 GHz and a lattice spacing, a =10 μm. By considering a generic vortex inducing pseudo-spin perturbation of strength κ′=0.1κ, we can estimate the interaction induced decay rate (equation (10)), Hz. As expected, such a decay rate is highly suppressed owing to the Majorana character of the edge-modes. For gaps on the order of GHz, dynamical decoherence typically yields a decay rate, kHz (refs 29 , 30 , 31 ). By gapping the dangling vortices associated with the edge, one can further suppress the noise spectral density of the bath and hence Γ dec p . Both decoherence rates are considerably smaller than those associated with current state of the art superconducting quantum channels [32] , [33] , [34] . With an edge velocity, m s −1 , the wavepacket’s edge traversal time (for mm) is t ∼ 0.1 μs, several orders of magnitude smaller than the decoherence induced decay times. In order to combine this unique pseudo-spin edge-channel with a long-lived quantum memory, we consider a hybrid architecture, involving three individual components: a spin-qubit memory, a pseudo-spin CSLB droplet and a mediating superconducting qubit (MSQ), which provides an interface between the spin memory and the SC-pseudo-spin edge modes [35] , [36] , [37] , [38] . An important source of infidelity arises from this MSQ interface. In order to map the quantum information from the spin memory to the pseudo-spin edge mode, we require the interaction strength between spin-MSQ to be larger than MHz (dephasing rate of the SC-qubit). However, the spin-MSQ coupling, which is naturally provided by the differing magnetic fields of the two persistent current quantum states of the SC-qubit, is estimated to be g ∼ 10 kHz [35] . To overcome this limitation, we envision using an off-resonant excitation scheme [35] . Within such a scheme, a natural optimum arises owing to an interplay between decoherence of the spin register ( ) and of the MSQ ( ); in particular, for an optimal detuning δ , one finds a minimal infidelity, . With experimentally accessible parameters, =1 μs and =10–100 ms, the optimized detuning becomes δ opt ≈1 MHz and yields ɛ opt ≪ 1% (refs 10 , 35 ). In addition, a channel composed from actual interacting spins can also be envisioned. Advances in atom-by-atom material design provide a promising avenue for the generation of complex atomic surface spin patterns [39] , [40] . Furthermore, tremendous progress in ion implantation suggests the possibility of fabricating lattice arrays of electronic spins as the basis for an in situ spin liquid [41] , [42] . One potential advantage of such an approach is the ability to harness the long coherence times associated with single-spin qubits [9] , [10] ; moreover, directly using solid-state spins also enables the manipulation, transfer and processing of quantum information usng the same fundamental hardware [43] . The search for novel topological phases represents one of the most exciting challenges in many-body physics; indeed, this challenge has led to a widespread effort to experimentally identify or engineer systems exhibiting exotic topological order. One of the prototypes of such order is provided by the CSLB phase of the Kitaev honeycomb model; although such chiral spin liquid phases have yet to be experimentally implemented, several realistic approaches towards their realization have been envisioned. For example, the realization of Kitaev’s gapped B phase is currently being considered in systems ranging from ultra-cold atoms [44] , [45] to polar molecules [46] , [47] . However, although recent experiments have demonstrated the ability to control ensembles containing tens of qubits [48] , [49] , [50] , such mesoscopic systems are insufficient in size to support the existence of several well-separated quasiparticles, a crucial prerequisite to demonstrate the non-abelian braiding essential for topological quantum computing [6] , [12] . By contrast, these smaller systems represent ideal candidates to demonstrate TPST and hence, the existence of a chiral fermion edge—another hallmark of the CSLB phase. Moreover, our proposed technique can also be used to directly characterize spin liquid states via passive spectroscopy of the droplet edge. By observing the splitting-dependent relaxation of the spin-qubit probe, one could map the energy spacing between the chiral edge modes. In addition, asymmetries in correlation measurements provide a direct indication of chirality. In this case, by gradually altering the physical distance separating two spin-qubit probes, one could characterize the timescale of incoherent interactions between the remote registers. Asymmetry in this timescale, dependent on the direction in which the qubits are separated provides a strong indication of the existence of a chiral edge and would enable direct evaluation of the velocity associated with the edge dispersion. Alternatively, one could also imagine holding the spin qubits fixed and characterizing asymmetries associated with L -to- R versus R -to- L TPST. These considerations imply that spin-qubit probes can provide a potential tool for exploring the properties of natural spin liquid candidates in both organic and inorganic insulators [15] , [51] , [52] , [53] . Spin-edge coupling and dangling vortices There are two types of excitations on the edge: Majorana fermions and vortices [17] . As the bulk phase is gapped, all static perturbations are irrelevant from a renormalization group point of view, with the low-energy effective edge theory remaining unchanged. Indeed, the topology of the bulk guarantees the existence of gapless chiral Majorana edge modes, as described by equation (8) [20] . Generically, all vortices are gapped; however, details of the lattice edge can lead to the existence of decoupled and/or low-energy vortices. Although the Hamiltonian in equation (8) does not capture these degrees of freedom, the presence of these additional states in the low-energy Hilbert space cannot be ignored. Indeed, the degeneracy of the exactly solved model follows from the presence of zero-energy dangling vortices formed by pairs of dangling Majoranas, as depicted in Supplementary Fig. S1 . Away from the injection point: (1) zero energy vortices are decoupled and hence irrelevant to TPST, (2) low-energy vortices scatter only weakly and (3) high-energy vortices are suppressed by temperature. The presence of a low-energy vortex degree of freedom at the injection point is critical to enable spin-edge coupling, which occurs at a dangling spin. Crucially, this dangling spin contains a decoupled, dangling Majorana operator ( Supplementary Fig. S1 ). Keeping track of this mode in the low-energy Hilbert space allows us to couple via . This is the continuum formulation of the microscopic coupling illustrated earlier. To further elucidate the importance of the vortex degree of freedom at the injection point, we consider three possibilities. First, in the case when the dangling injection Majorana is completely decoupled, the injection vortex (corresponding to the flipped U i , j at the injection point) is zero energy and the procedure for TPST remains identical. Second, in the case when the injection Majorana is weakly interacting with a single nearby Majorana (respecting the interaction symmetry), the injection vortex is low energy. In this case, the splitting of the spin register will need to be retuned to account for the creation of this low-energy vortex and TPST will then naturally create both a fermion and an injection vortex. Crucially, tunnelling of the injection vortex into the bulk will be energetically disallowed as . Problems only arise in the third case, when the injection Majorana is interacting strongly (order κ) with a single nearby Majorana, and the injection vortex is hence high energy. In this case, spin-edge coupling will create an injection vortex, which can diffuse into the bulk; thus, upon the return of the travelling fermion, the injection vortex may no longer be localized near the injection point, causing dephasing when the quantum information is recaptured. Suppressed interactions on the chiral edge Here, we consider the role of interactions between edge modes. The fidelity of topological state transfer will be dependent on these interactions as they induce decay of the Majorana quasiparticles. Here, we begin by estimating the lifetime of such excitations in the continuum edge setting by taking into account the leading order interaction term. We consider, at T =0, the situation where we tunnel a single-quasiparticle excitation into the chiral edge from an associated spin register. The Hamiltonian characterizing the Majorana edge and its leading order interaction is H = H e + H′ e . To evaluate the interaction induced decay rate of the quasiparticles, we use Fermi’s golden rule and consider the relevant interaction matrix elements coupling an incoming excitation γ p |Ω〉 with three outgoing (decayed) excitations . The associated decay rate takes the form, where the δ-function imposes energy conservation and the integrals are 1D, because the quasiparticle is confined to the droplet edge. To evaluate the decay rate, we begin by considering the interaction matrix element, where we have represented the interaction Hamiltonian in momentum space; by using Wick’s theorem, we can contract the matrix element into a function of two point Majorana correlators. The only terms from this contraction that contribute are connected terms of the form and such terms yield Γ ∼ λ 2 p 13 / ν . The leading order temperature correction in the limit | νp | ≫ kT is obtained from a Sommerfeld-type expansion [54] and yields equation (10). How to cite this article: Yao, N. Y. et al. Topologically protected quantum state transfer in a chiral spin liquid. Nat. Commun. 4:1585 doi: 10.1038/ncomms2531 (2013).